Homoepitaxial tunnel barriers with functionalized graphene-on-graphene for charge and spin transport The coupled imperatives for reduced heat dissipation and power consumption in high-density electronics have rekindled interest in devices based on tunnelling. Such devices require mating dissimilar materials, raising issues of heteroepitaxy, layer uniformity, interface stability and electronic states that severely complicate fabrication and compromise performance. Two-dimensional materials such as graphene obviate these issues and offer a new paradigm for tunnel barriers. Here we demonstrate a homoepitaxial tunnel barrier structure in which graphene serves as both the tunnel barrier and the high-mobility transport channel. We fluorinate the top layer of a graphene bilayer to decouple it from the bottom layer, so that it serves as a single-monolayer tunnel barrier for both charge and spin injection into the lower graphene channel. We demonstrate high spin injection efficiency with a tunnelling spin polarization >60%, lateral transport of spin currents in non-local spin-valve structures and determine spin lifetimes with the Hanle effect. The quantum phenomenon of tunnelling enables novel charge-based devices with ultra-low power consumption [1] , and is key to the emerging field of spintronics [2] , [3] . Tunnel devices typically require mating dissimilar materials and maintaining monolayer level control of thickness, raising issues that severely complicate fabrication and compromise performance. The recent discoveries of intrinsically two-dimensional (2D) materials [4] , such as graphene and h-BN have created new perspectives on tunnel barriers [5] , [6] , [7] , [8] . Their strong in-plane bonding promotes self-healing of pinholes [9] and a well-defined layer thickness, important because the tunnel current depends exponentially on the barrier thickness. There has been keen interest in utilizing graphene, a 2D honeycomb lattice of carbon atoms, as a high-mobility transport channel. Its linear band dispersion, ambipolar conduction and remarkable in-plane electronic transport properties [10] have stimulated development of RF transistors and wafer-scale fabrication of graphene circuits [11] . Graphene also exhibits exceptional in-plane spin transport characteristics, including long spin diffusion lengths owing to its low spin–orbit interaction [12] , [13] , [14] , which has stimulated ideas for novel spin devices [15] . The highest values for charge mobility, spin diffusion lengths and spin lifetimes have been measured using mechanically exfoliated graphene. However, exfoliated graphene is not amenable for general device fabrication and scalability, because devices must be fabricated on individual, randomly placed and sized flakes. Moreover, spin injection into graphene from a ferromagnetic (FM) metal contact typically requires the use of an oxide tunnel barrier, such as Al 2 O 3 (ref. 12 ) or MgO (ref 13 ), to accommodate the large conductivity mismatch [16] , [17] . These materials do not wet the graphene surface, making it very difficult to control the thickness and uniformity of the tunnel barrier. In addition, the mobility of graphene is significantly degraded by coupling to phonons or charged impurities/defects in an adjacent oxide. Consequently, significant effort has focused on exploiting other carbon-thin films and 2D materials such as h-BN or MoS 2 as a substrate, gate dielectric or tunnel barrier for graphene devices [7] , [8] , [10] , [18] , [19] . This improves operating characteristics, but significantly complicates the fabrication, and often relies on sequential mechanical exfoliation to produce a few device structures. Although single-layer graphene itself has been shown to function as a tunnel barrier in a heterostructure [5] , [6] , [20] , [21] , it does not effectively serve as a tunnel barrier on another layer of graphene because there is always some electrical interaction between the two layers, regardless of the stacking orientation [22] , [23] , except in a large magnetic field [24] . One can markedly alter graphene’s physical properties with chemical functionalization [25] . Fluorinated graphene is an excellent in-plane insulator, and no electrical communication is observed between adjacent layers of fluorographene and graphene [23] , suggesting its use as a tunnel barrier in an all-graphene tunnel-transport homoepitaxial structure. Here, we show that relatively complex charge/spin transport device structures, such as the non-local spin valve (NLSV), can be fabricated using graphene both as the transport channel as well as the tunnel barrier, obviating the need for the growth of a separate dielectric material. We fabricate spin devices where a monolayer of fluorinated graphene acts as a tunnel barrier on a monolayer of non-functionalized graphene, and demonstrate electrical spin injection, lateral transport and detection by a four-terminal (4T) NLSV and Hanle effect measurements. We find the highest spin efficiency values yet measured for graphene, and present evidence for the theoretically predicted enhancement of tunnel spin polarization [21] . Furthermore, the gate voltage dependence of the spin lifetime and spin signal indicates that fluorinated graphene tunnel barriers allow a better sampling of graphene’s intrinsic spin properties than with most oxide tunnel barriers. Fluorographene/graphene enables realization of homoepitaxial, few-layer carbon structures for versatile electronic devices, such as magnetologic gates [15] . Charge tunnelling through fluorinated graphene Schematic and optical images of the NLSV devices used in this work are shown in Fig. 1a,b , respectively. The structures consist of two FM permalloy/fluorinated graphene tunnel contacts (contacts 2 and 3, shown in red) placed between two Au/Ti contacts (contacts 1 and 4, shown in gold). Details of fabrication and measurement are found in the Methods, Supplementary Methods , Supplementary Fig. 1 and Supplementary Fig. 2 . The Au/Ti contacts show Ohmic behaviour, as expected. The conductance versus back gate voltage, measured between the two Ohmic Au/Ti contacts ( Fig. 2a , black curve), shows the Dirac point of the bottom graphene channel at ~80 V, indicating a high electron concentration. The high doping level is most likely due to extrinsic residues and charging in the SiO 2 substrate resulting from device processing. The transistor characteristics measured between the two permalloy (Py, Ni 80 Fe 20 ) contacts that only contact the top fluorinated graphene film ( Fig. 2a , blue curve), show no modulation or Dirac point. This confirms that the graphene layers are indeed not communicating electrically, as expected after fluorination. The conductance of the device between these two Py contacts is orders of magnitude less than the conductance of the fluorinated graphene film, indicating that all of the electrical transport measured is due to tunnelling through the fluorinated graphene and into the underlying graphene transport channel. 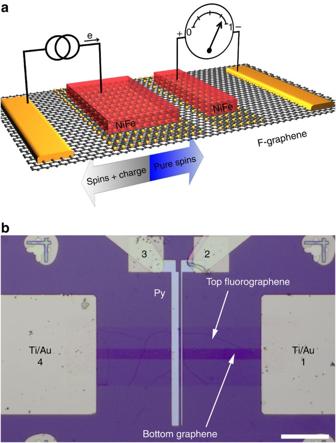Figure 1: The homoepitaxial tunnel barrier device. (a) Schematic and (b) optical image of a typical device. Scale bar, 20 μm. Here, the left permalloy (NiFe, Py) contact is 3 μm wide and separated from the right Py contact (500 nm wide) by 1 μm. We number the contacts 1 to 4 from right to left. Figure 1: The homoepitaxial tunnel barrier device. ( a ) Schematic and ( b ) optical image of a typical device. Scale bar, 20 μm. Here, the left permalloy (NiFe, Py) contact is 3 μm wide and separated from the right Py contact (500 nm wide) by 1 μm. We number the contacts 1 to 4 from right to left. 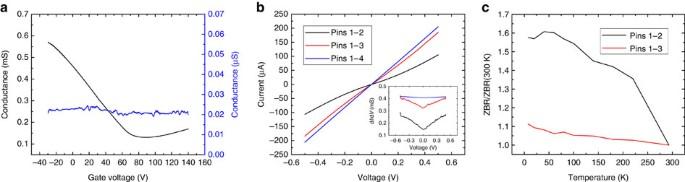Figure 2: Charge transport data. (a) Dirac curves taken using the SiO2/Si substrate as a back gate. Blue: between contacts 2 and 3 (only on the fluorographene). Black: between contacts 1 and 4 (only on the graphene channel). The fluorographene shows no Dirac point, indicating that it is fully insulating and electrically uncoupled from the graphene that is underneath it. (b) current-voltage curves for a typical device. Taken between contacts 1 and 2 or 1 and 3 (includes the tunnel barrier), the curves are non-Ohmic. Taken between contacts 1 and 4 (graphene channel only) the curve is linear. The inset further highlights this by showing dV/dIversusVwhen the tunnel barrier is included in the circuit. (c) Zero bias resistance versus temperature for the Py contacts showing a weak temperature dependence (non-metallic behaviour) that is a hallmark of a good tunnel barrier. Full size image Figure 2: Charge transport data. ( a ) Dirac curves taken using the SiO 2 /Si substrate as a back gate. Blue: between contacts 2 and 3 (only on the fluorographene). Black: between contacts 1 and 4 (only on the graphene channel). The fluorographene shows no Dirac point, indicating that it is fully insulating and electrically uncoupled from the graphene that is underneath it. ( b ) current-voltage curves for a typical device. Taken between contacts 1 and 2 or 1 and 3 (includes the tunnel barrier), the curves are non-Ohmic. Taken between contacts 1 and 4 (graphene channel only) the curve is linear. The inset further highlights this by showing d V /d I versus V when the tunnel barrier is included in the circuit. ( c ) Zero bias resistance versus temperature for the Py contacts showing a weak temperature dependence (non-metallic behaviour) that is a hallmark of a good tunnel barrier. Full size image Figure 2b shows IV curves taken between the Py and the Ohmic Au/Ti contacts. These curves exhibit markedly non-Ohmic behaviour, further emphasized in the inset of Fig. 2b with a graph of the differential conductance versus voltage, and provide additional support that the fluorinated graphene is acting as a tunnel barrier. The temperature dependence of the zero bias resistance ( Fig. 2c ) is weak and insulator-like in character, changing by a factor less than 1.7 for both Py contacts. Non-Ohmic IV curves and a weak temperature-dependent zero bias resistance has been shown to be a firm confirmation of tunnelling behaviour in the contacts [26] . Spin injection and lateral transport In NLSV measurements [27] , a bias current is applied between one of the FM contacts and the nearest Ohmic reference contact, and a spin-polarized charge current is injected from the FM across the fluorinated graphene tunnel barrier and into the graphene transport channel. This spin-charge current follows the electric field and flows as shown in Fig. 1a . Spin simultaneously diffuses in all directions, creating a pure spin current, and the corresponding spin accumulation results in a spin-splitting of the chemical potential. This is manifested as a voltage on the second FM contact, which is outside of the charge current path and referred to as the non-local detector. An in-plane magnetic field is used to control the relative orientation of the magnetizations of the FM injector and detector contacts. When the magnetizations are parallel, the voltage measured will be smaller than when they are antiparallel. Sweeping the magnetic field causes the contact magnetizations to reverse in-plane at their respective coercive fields and produce a measurable voltage peak. In order to observe this effect, we fabricate the Py contacts with two different widths (0.5 and 3 μm) to exploit magnetic shape anisotropy so that the coercivities of the FM contacts are different. This NLSV behaviour is clearly observed in Fig. 3a , where distinct steps in the non-local resistance (the measured voltage divided by the bias current) appear at the coercive fields of the wide and narrow FM contacts, producing plateaus of higher resistance when the FM contact magnetizations are antiparallel. This demonstrates successful spin injection and detection at the FM/fluorinated graphene tunnel contacts, and lateral spin transport in the graphene channel. 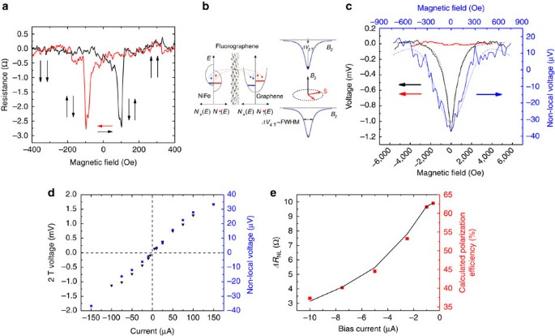Figure 3: Spin transport data. (a) NLSV measurement. The horizontal arrows indicate the direction of the field sweep. The vertical arrows indicate the FM magnetization directions. A small constant background of ~400 Ohms was subtracted from the data. (b) Energy diagram showing how spins tunnel from the permalloy (NiFe, Py) across the fluorographene and into the graphene channel. Theoretical Hanle curves for 2T and 4T measurements are depicted on the right. (c) 4T Hanle (blue, top and right axes) versus 2T Hanle and witness sample (black/red, bottom and left axes). The dotted lines show fits to the appropriate models. Here,τsfor 2T/4T was 96 ps/205 ps, respectively. (d) Bias dependence of 2T (black triangle) and 4T (blue square) Hanle signal amplitude. (e) Bias dependence of the NLSV plateauΔRNLand the spin polarization efficiency, showing strong evidence of spin-filtered tunneling. Figure 3: Spin transport data. ( a ) NLSV measurement. The horizontal arrows indicate the direction of the field sweep. The vertical arrows indicate the FM magnetization directions. A small constant background of ~400 Ohms was subtracted from the data. ( b ) Energy diagram showing how spins tunnel from the permalloy (NiFe, Py) across the fluorographene and into the graphene channel. Theoretical Hanle curves for 2T and 4T measurements are depicted on the right. ( c ) 4T Hanle (blue, top and right axes) versus 2T Hanle and witness sample (black/red, bottom and left axes). The dotted lines show fits to the appropriate models. Here, τ s for 2T/4T was 96 ps/205 ps, respectively. ( d ) Bias dependence of 2T (black triangle) and 4T (blue square) Hanle signal amplitude. ( e ) Bias dependence of the NLSV plateau ΔR NL and the spin polarization efficiency, showing strong evidence of spin-filtered tunneling. Full size image Spin lifetime and the Hanle effect The spin lifetime corresponding to this pure spin current is quantitatively determined using the Hanle effect [3] , [6] , in which a magnetic field B z applied along the surface normally causes the spins in the graphene transport channel to precess at the Larmor frequency, ω L = gμ B B z / ħ , and dephase, as illustrated in Fig. 3b . Here g is the Lande g -factor ( g ~2 for graphene), μ B is the Bohr magneton and ħ is Planck’s constant. As the magnetic field increases, the net spin polarization and corresponding spin voltage decreases to zero with a characteristic pseudo-Lorentzian line shape. Figure 3c shows Hanle spin precession curves for both non-local (blue) and local (black) contact geometries for a typical device used in this study in comparison with a witness sample device, where the top graphene layer was not fluorinated (red curve). We note that no NLSV signal or Hanle effect is apparent in the witness sample, demonstrating that the fluorinated graphene tunnel barrier is necessary to achieve spin injection. We measure Hanle spin precession in two different electrical configurations. The spin lifetime of the pure spin current is measured in the NLSV or 4T configuration, where the full-width-half-max of the measured change in voltage is directly proportional to the steady-state spin polarization at the detector, given by [3] where spin is injected into the graphene at x 1 and t= 0 and detected at x 2 . S 0 is the spin injection rate, D is the electron diffusion constant, v d is the electron drift velocity (=0 for diffusive transport) and τ s is the spin lifetime. Second, the spin current can be injected and the spin voltage detected with the same Py contact in a two-terminal (2T) configuration. Here, we measure the spin accumulation and lifetime directly under the Py contact, and the voltage ΔV 2T ( B z ) decreases with B z with a Lorentzian line shape given by ΔV 2T ( B z )= ΔV 2T (0)/[1+( ω L τ s ) 2 ] (ref. 6 ). In this way, fits to the Hanle curves allow us to extract the spin lifetime (for the 2T and 4T case) and the spin diffusion constant (for the 4T case). In Fig. 3c , we see a strong Hanle signal from the 4T non-local measurement (blue curve) and the 2T measurement (black curve). The Hanle signal persists up to ~200 K. Average 4T spin lifetimes were ~200 ps and average 2T spin lifetimes were ~100 ps. We attribute the shorter spin lifetime to increased scattering and depolarization that occur at the Py contact interface relative to that in the lateral graphene transport channel. The spin diffusion length is given by L SD =( Dτ s ) 1/2 , where D is the diffusion constant [3] . We find an average L SD ~ 1.5 μm, based on τ s ~ 200 ps and D ~0.01224, m 2 s −0 consistent with other studies of chemical vapour deposition (CVD)-grown graphene films [28] . Although CVD-grown graphene does not match the electrical properties of mechanically exfoliated graphene, it is amenable to industrial-scale fabrication, and, as fabrication methods are honed (see Supplementary Methods and Supplementary Fig. 1 ), we expect the properties of the two types of graphene to converge. Figure 3d shows the bias dependence of the magnitude of the 4T non-local and 2T Hanle voltage taken at B =0. Both are approximately linear with bias current, as expected. The observation of both the non-local Hanle effect and the NLSV provides strong evidence that the fluorinated graphene tunnel barrier indeed enables efficient spin injection, transport and detection in the graphene channel. Tunnelling spin polarization On the basis of magnitude of the NLSV signal ( Fig. 3a ) and the calculated spin diffusion length from the 4T Hanle measurements, we can determine the tunnelling spin polarization, P , of the Py/fluorinated graphene contact using the formula [12] : where σ is the measured conductivity of 1.29 × 10 −4 Ω −1 for the device shown in Fig. 3a , L is the centre-to-centre contact spacing of 5.75 μm, L SD is the spin diffusion length of 1.5 μm, W is the width of the graphene channel of 5 μm and ΔR NL ~3 Ω is the magnitude of the NLSV plateau for a bias current of −10 μA. From this, we find P ~35%. Fig. 3e summarizes the bias dependence ΔR NL and P . Both increase monotonically with decreasing bias, typical of graphene NLSV devices [12] , [13] . In contrast with previous work, we measure values of P up to ~63% at low bias, significantly higher than both the intrinsic spin polarization of Ni 80 Fe 20 and the values of 32–48% reported in the literature for the tunnelling spin polarization of Ni 80 Fe 20 /Al 2 O 3 tunnel barriers [29] . This value is also much larger than the highest values measured to date ( P =26–30%) in graphene NLSV devices with alumina or MgO tunnel barriers [12] , [13] . This indicates that significant spin filtering occurs at the Py/fluorinated−graphene interface, consistent with theoretical predictions for spin transport across Ni/graphene lattice-matched interfaces [21] , and is the first demonstration of enhanced tunnelling spin polarization in a graphene-based tunnel structure. The non-linear increase of polarization as the bias current approaches zero is consistent with other spin valve studies, although it is not entirely understood [6] . To better compare our results with theory and evaluate the performance of the fluorinated tunnel barrier, we calculate the spin resistance-area (RA) product, ΔV 2T (B =0 )A/I b , where A is the contact area and I b is the bias current. For the device shown in Fig. 3 , we measure a spin RA product of 30 Ω μm 2 . The theoretical spin RA product is given by γ 2 ρL sd W/w , where W is the channel width and w is the thickness [16] . Using a tunnelling spin polarization value γ=P ~0.35 measured at this bias, we calculate the theoretical spin RA product to be ~31 Ω μm 2 . The high tunneling spin polarization that we determine and the excellent agreement between our measured spin RA product and the theoretical value provide further evidence for the efficacy of the fluorinated graphene tunnel barrier. 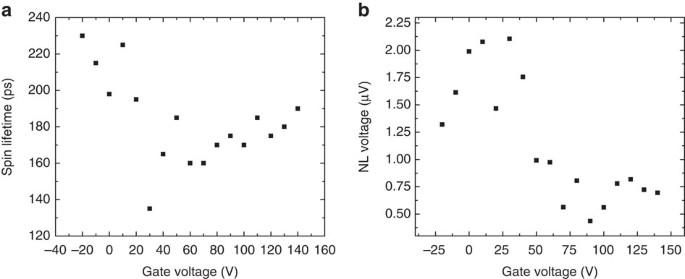Figure 4: Gate voltage dependence of spin transport. Gate voltage dependence for (a) 4T spin lifetime and (b) 4T Hanle magnitude. The bias current was −10 μA. Figure 4a,b shows the dependence of the 4T Hanle spin lifetime and signal amplitude on gate voltage. We see a dependence that resembles the Dirac curve (in Fig. 2a ). Both parameters increase with increasing carrier density, with the effect more pronounced for whole density. Theory predicts that the spin lifetime will increase with increased carrier density owing to a decreasing correlation length of the Rashba spin-orbit coupling field (induced through interaction with the substrate), and thus decreased spin-flip scattering [30] . Others have suggested a completely different spin relaxation mechanism arising from resonant spin scattering by local magnetic moments at vacancy or adatom sites, and predict an increase of spin lifetime with carrier density, as we observe in Fig. 4a (ref. 31 ). However, the dominant spin relaxation mechanism in graphene remains unclear. Figure 4: Gate voltage dependence of spin transport. Gate voltage dependence for ( a ) 4T spin lifetime and ( b ) 4T Hanle magnitude. The bias current was −10 μA. Full size image While most early graphene spin experiments showed spin lifetimes that are constant in gate voltage [12] , other work shows that spin lifetimes are affected by changes in carrier density [32] . Studies that observe gate voltage dependence have in common high contact resistance in the oxide tunnel barrier contacts, indicative of pinhole-free tunnel barriers that prevent back diffusion into the FM contact and subsequent fast spin relaxation [33] . The discrepancy between these measurements is thus likely related to differences in the quality of the tunnel barrier contacts. Oxide tunnel barriers are known to be very difficult to form on graphene since they exhibit de-wetting in the absence of prior chemical treatment of the graphene, and attempts to mitigate this to create a good surface for oxide growth may induce scatterers and defects [34] . Thick oxide tunnel barriers can also irreversibly structurally damage graphene [35] . In all of these cases, it would be difficult to measure the intrinsic properties of the graphene itself. The single-atom thick fluorinated graphene tunnel barrier offers an elegant solution. Our experiments show a clear gate voltage-dependent spin signal that follows the Dirac curve, just as predicted by theory. In conclusion, we have demonstrated a unique homoepitaxial tunnel barrier system in which graphene serves as both the tunnel barrier and the high-mobility transport channel. Our measurements show that fluorination of the upper layer in a graphene bilayer film creates an effective tunnel barrier for spin injection and detection in the lower graphene channel. NLSV and corresponding Hanle measurements attest to the quality of these devices. In contrast with most oxide tunnel barriers on graphene, fluorinated graphene provides much larger tunnelling spin polarization efficiency that we attribute to interface spin filtering, a more uniform and well-controlled barrier, and allows the observation of the theoretically predicted Hanle voltage and spin lifetime on gate voltage. Fluorographene/graphene enables realization of homoepitaxial few-layer carbon structures for versatile electronic devices. Graphene growth Graphene is grown by CVD on Cu foil [36] , and a single layer transferred to a 275 nm SiO 2 /Si substrate. Additional details can be found in the Supplementary Methods and Supplementary Fig. 1 . Device fabrication Electron-beam lithography with an MMA/PMMA resist layer is used to protect rectangular strips of graphene and the excess is burned away in O 2 plasma, defining the graphene spin channel mesas. Ohmic Ti/Au contacts (5/35 nm thick) are fabricated by electron-beam lithography and electron-beam evaporation. A second layer of CVD graphene is then transferred onto the structures and the same method described above is used to define mesas in this second layer, which completely overlaps the underlying graphene channel. Channels are opened in an MMA/PMMA layer for the FM contacts, and the graphene exposed by these channels is fluorinated in XeF 2 gas to a resistance of 50 GΩ, as measured by a concurrently fluorinated two-electrode witness device. Permalloy (Py, Ni 80 Fe 20 ) is then deposited by electron-beam evaporation directly followed by a thin Au capping layer, to form contacts 3 and 0.5 μm wide, separated by 1 or 4 μm. After lift-off, a final XeF 2 gas exposure fluorinates the remaining portions of the top graphene layer not covered by the Py contacts to a resistance of 50 GΩ just before electrical measurement, ensuring that no parallel conductance paths exist, and eliminating possible edge state conduction and possible magnetic effects [37] , [38] . Further sample fabrication details can be found in the Supplementary Methods and Supplementary Fig. 2 . Device measurement Magnetotransport measurements are performed in a cryogen-free, variable temperature (10–300 K) cryostat and electromagnet assembly. How to cite this article: Friedman, A. L. et al . Homoepitaxial tunnel barriers with functionalized graphene-on-graphene for charge and spin transport. Nat. Commun. 5:3161 doi: 10.1038/ncomms4161 (2014).